Plant cysteine oxidases control the oxygen-dependent branch of the N-end-rule pathway In plant and animal cells, amino-terminal cysteine oxidation controls selective proteolysis via an oxygen-dependent branch of the N-end rule pathway. It remains unknown how the N-terminal cysteine is specifically oxidized. Here we identify plant cysteine oxidase (PCO) enzymes that oxidize the penultimate cysteine of ERF-VII transcription factors by using oxygen as a co-substrate, thereby controlling the lifetime of these proteins. Consequently, ERF-VII proteins are stabilized under hypoxia and activate the molecular response to low oxygen while the expression of anaerobic genes is repressed in air. Members of the PCO family are themselves targets of ERF-VII transcription factors, generating a feedback loop that adapts the stress response according to the extent of the hypoxic condition. Our results reveal that PCOs act as sensor proteins for oxygen in plants and provide an example of how proactive regulation of the N-end rule pathway balances stress response to optimal growth and development in plants. Adequate provision of oxygen to sustain aerobic metabolism is not always guaranteed throughout a plant’s lifecycle. In fact, hypoxic conditions may arise because of reduced oxygen levels in the environment, sudden increase of the respiratory demand or endogenous barriers to oxygen diffusion [1] . The resulting reduced availability of oxygen can cause decreased energy production via oxidative phosphorylation and limits any other reaction that uses oxygen as substrate as well. Consequently, development [2] and growth [3] , [4] are affected and plant survival is jeopardized if cells do not react promptly [5] . Oxygen sensing in plants is mediated by a branch of the amino-end rule pathway that controls the stability of the constitutively expressed ERF-VII transcription factor RAP2.12 and its homologue RAP2.2, which are primary activators of the anaerobic response genes [6] . The N-end rule pathway describes a series of reactions that controls proteins’ degradation depending on the nature of their N-terminal residue [7] , [8] . Primary destabilizing amino acids (Arg, His and Lys) specify sequences, defined as degrons, which are recognized by single subunit E3 ubiquitin ligases (called PRT in plants or UBR in animals) that direct substrate proteins towards degradation via the 26S proteasome [8] . Secondary destabilizing residues (Asp, Glu or oxidized Cys) function as substrates for arginyl-transfer RNA transferases (ATE) to conjugate a primary destabilizing Arg residue [8] . Finally, tertiary destabilizing residues (Gln, Asn and Cys) require chemical modifications to generate secondary destabilizing amino acids. In any case, to act as destabilizers all these residues have to be exposed at the N terminus of proteins either via Met-aminopeptidases that remove the initial methionine [9] , or via selective cleavage by endoproteases. The Cys branch of the N-end rule pathway involves the oxygen-dependent oxidation of N-terminal Cys residues to Cys sulphinic acid (CSA) or Cys sulphonic acid [6] , [10] , [11] . In plants, the occurrence of an N-terminal Cys residue was shown to be essential to generate a functional degron in the ERF-VII proteins and other transcription factors [11] . Despite its importance to initiate the Cys branch of the N-end rule during developmental processes and stress response [1] , [12] , it remained unresolved how the oxidation of the N-terminal Cys of a protein is mediated to adjust the cellular response to oxygen availability. In animals, N-terminal Cys sulphinic or -sulphonic acid is assumed to be spontaneously formed in the presence of strong oxidants such as hydrogen peroxide and nitric oxide (NO) [13] . However, exclusive control by spontaneous redox-driven reactivity of the initiation of the anaerobic response in plants would expose oxygen perception to uncontrolled variations of the redox status of the cells. In addition, it would impair fine-tuning mechanisms, such as those observed for the primary activator of the anaerobic response hypoxia inducible factor 1-α (HIF1-α) in animal cells [14] . In this system, amino acid-hydroxylase enzymes use oxygen as co-substrate to control the stability and activity of HIF1-α [15] , thereby enabling the cell to modulate the response to oxygen limitation. In this perspective, it would seem limiting for plant cells to rely merely on a spontaneous reaction to perceive oxygen availability, while the existence of enzymatic catalysis would positively contribute to successful adaptation. In this study, we report the identification and functional characterization of a novel class of enzymes in the plant Arabidopsis thaliana , which we named plant cysteine oxidases (PCOs). Knocking out two of the most expressed PCO genes is sufficient to induce the core set of hypoxia-response genes under aerobic conditions, while overexpression of PCO1 or PCO2 suppresses the induction of these genes in hypoxia. We show that PCO proteins facilitate the oxidation of N-terminal cysteine residues to CSA using molecular oxygen as a co-substrate, thus preparing the protein for N-end rule pathway-mediated proteasomal degradation. By using a combination of stably transformed plants and transient expression in protoplasts, we demonstrate that the effect of PCOs on the molecular response to hypoxia involves RAP2.12 and is independent of its DNA-binding properties. In addition, PCO1 and PCO2 are induced by RAP2.12, thereby generating a feedback loop that enables homoeostatic control of the anaerobic response. We also show that alterations of their expression pattern compromise the ability of Arabidopsis to endure submergence. In conclusion, we demonstrate that PCOs are involved in the N-end rule pathway-mediated proteolysis and control the preparation of ERF-VII proteins for degradation via the 26S proteasome. This discovery highlights the evolutionary convergence of the oxygen-sensing mechanisms in animals and plants, both of them based on the enzymatic control of the stability of transcriptional regulators that mediate the response to oxygen limitations. PCOs oxidize N-terminal cysteine to CSA Searching for enzymes putatively involved in the oxidation of N-terminal Cys, we identified a gene family conserved among plants, with five members in A. thaliana, encoding proteins that share a conserved domain present in thiol -oxidases such as animal cysteine and cysteamine dioxygenase ( Supplementary Fig. 1 ) [16] . N-terminal fusion of members of this protein family to enhanced green fluorescent protein (GFP) revealed that PCOs are localized in both the cytosol and nucleus of plant cells ( Fig. 1a ). When purified after heterologous expression in Escherichia coli , the proteins exhibited cysteine sulphinic acid (CSA) synthetase activity ( Fig. 1b ) using cysteine and oxygen as substrates ( Fig. 1b,c ). Therefore, we called them PCOs. Interestingly, PCO1 and PCO2 activities were two- to fivefold higher when Cys was the N-terminal amino-acidic residue of a peptide ( Fig. 1c , Supplementary Fig. 2a ), while Cys was not oxidized by PCO1 when the residue was located inside or at the C terminus of a peptide ( Supplementary Fig. 2b ). PCOs could not oxidize internal Cys even in a peptide known to possess an oxidation-prone Cys residue, such as the one corresponding to the regulatory Cys149 of the subunit 1 of the cytosolic glyceraldehyde-3-phosphate dehydrogenase of Arabidopsis [17] ( Fig. 1c ). 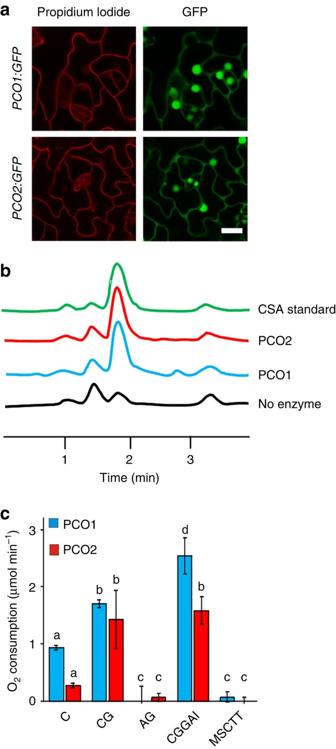Figure 1: The plant cysteine oxidase(PCO)genes encode for cytosolic and nuclear enzymes that oxidize N-terminal cysteine residues in peptides. (a) Subcellular localization of PCO1 and PCO2. Scale bars, 10 μm. (b) HPLC detection of Cys sulphinic acid (CSA) production via oxidation of cysteine in absence (black) or presence of purified PCO1 (blue), PCO2 (red) proteins. The retention time of a CSA standard is shown in green. (c) Oxygen consumption by PCO1 and PCO2 in a Cys oxidationin vitroassay using free cysteine (C), CG and AG dipeptide or CGGAI and MSCTT pentapeptides. Data are presented as mean±s.d. (n=6). Letters indicate statistically significant difference (P<0.05, two-way analysis of variance) for each enzyme separately. Figure 1: The plant cysteine oxidase (PCO) genes encode for cytosolic and nuclear enzymes that oxidize N-terminal cysteine residues in peptides. ( a ) Subcellular localization of PCO1 and PCO2. Scale bars, 10 μm. ( b ) HPLC detection of Cys sulphinic acid (CSA) production via oxidation of cysteine in absence (black) or presence of purified PCO1 (blue), PCO2 (red) proteins. The retention time of a CSA standard is shown in green. ( c ) Oxygen consumption by PCO1 and PCO2 in a Cys oxidation in vitro assay using free cysteine (C), CG and AG dipeptide or CGGAI and MSCTT pentapeptides. Data are presented as mean±s.d. ( n =6). Letters indicate statistically significant difference ( P <0.05, two-way analysis of variance) for each enzyme separately. Full size image PCO1 and PCO2 are hypoxia-inducible genes To evaluate the biological role of PCO1 and PCO2, we analysed their expression pattern using Genevestigator [18] . All PCO genes were expressed at medium level throughout plant development ( Fig. 2a , Supplementary Table 1 ) while PCO1 and PCO2 were also specifically induced by oxygen shortage ( Fig. 2b ). Indeed, both genes are listed as part of the core molecular response to hypoxia [19] and are suggested to be directly controlled by the interaction of RAP2.12 with an ATCTA element present in their promoter [6] ( Supplementary Fig. 3 ). Fusion of the promoter of PCO1 and PCO2 with a GUS:GFP reporter confirmed the induction of these two proteins in Arabidopsis seedlings by oxygen deprivation ( Fig. 2c ). Throughout development, the expression of PCO1 and PCO2 genes was highest in mature siliques and during seed germination ( Fig. 2a ), two conditions that are characterized by low oxygen availability [20] . Taken together, our expression analysis clearly suggests a role of PCOs in the stress response of plants to hypoxia. 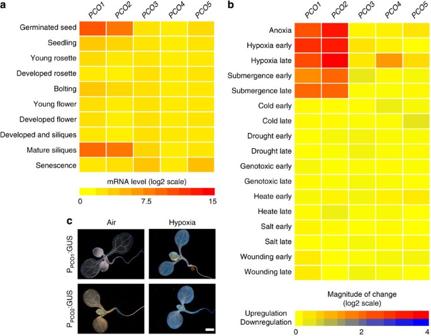Figure 2:PCO1andPCO2are specifically induced oxygen deficiency. (a) Expression ofPCO1andPCO2genes throughout development inA. thaliana.Numeric expression values are shown inSupplementary Table 1. (b) Stress-related messenger RNA expression level of the fivePCOgenes. Expression data were exported from the Genevestigator20database choosing the experimental data set that best represented an average of the conditions considered. (c) Spatial visualization ofPCO1andPCO2promoter activity by GUS-reporter staining. Scale bar, 1 mm. Figure 2: PCO1 and PCO2 are specifically induced oxygen deficiency. ( a ) Expression of PCO1 and PCO2 genes throughout development in A. thaliana. Numeric expression values are shown in Supplementary Table 1 . ( b ) Stress-related messenger RNA expression level of the five PCO genes. Expression data were exported from the Genevestigator [20] database choosing the experimental data set that best represented an average of the conditions considered. ( c ) Spatial visualization of PCO1 and PCO2 promoter activity by GUS-reporter staining. Scale bar, 1 mm. Full size image PCO1 and PCO2 redundantly repress the anaerobic response To investigate the effect of PCOs on the Arabidopsis transcriptome, we carried out a microarray-based analysis of PCO1 -overexpressing plants. By using a selection of three independent transgenic lines that did not exhibit strong alteration in growth and development, we avoided the identification of differentially expressed genes (DEGs) that would arise from secondary effects. Overall, a small number of genes exhibited a significant alteration of at least twofold in PCO1 -overexpressing lines as compared with wild-type: 21 DEGs under aerobic conditions and 22 under hypoxia, respectively ( Supplementary Tables 2 and 4 ). About 90% of the DEGs in air were downregulated in 35S:PCO1 plants ( Supplementary Table 2 ). 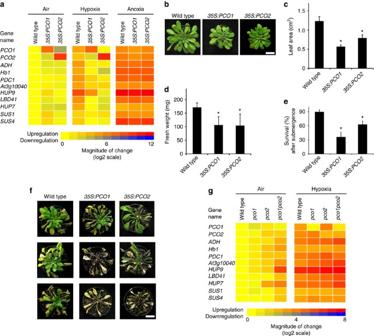Figure 3: PCO1 and PCO2 redundantly repress the molecular response to hypoxia, thereby reducing tolerance to submergence. (a) Differential expression of hypoxia-responsive genes inPCO-overexpressing plants as compared with wild-type under aerobic, hypoxic or anoxic conditions (reference: wild-type in air,n=5). Numeric expression values and statistical significance are shown inSupplementary Table 6. (b) Phenotype ofPCO1- andPCO2-overexpressing plants; scale bar, 2 cm. (c) Leaf area of wild type and35S:PCO1and35S:PCO2plants. Data are presented as mean±s.d. (n=5). Asterisks indicate statistically significant difference from wild type (P<0.05, one-way analysis of variance (ANOVA)). (d) Dry weight of wild-type andPCO-overexpressing plants. Data are presented as mean±s.d. (n=10).Asterisks indicate statistically significant difference from wild type (P<0.05, one-way ANOVA). (e) Percentage of PCO overexpressors and wild-type plants surviving flooding-induced hypoxia. Data are presented as mean±s.d. (n=4). Asterisks indicate statistically significant difference from wild type (P<0.05, one-way ANOVA). (f) Phenotypes of wild-type,35S:PCO1and35S:PCO2plants recovering from dark submergence (72 h). Scale bar, 2 cm. (g) Heatmap depicting the expression of hypoxia-inducible genes inpco1-,pco2-andpco1pco2-double mutant plants as compared with the wild type under aerobic and hypoxic conditions (reference wild type in air,n=4). Numeric expression values and statistical significance are shown inSupplementary Table 7. Among these genes, over 30% corresponded to genes known to be induced by hypoxia and 50% to genes upregulated during germination ( Supplementary Table 3 ). Under hypoxic conditions, this pattern was further highlighted: over 80% of the genes downregulated in 35S:PCO1 plants as compared with the wild type are hypoxia inducible ( Supplementary Fig. 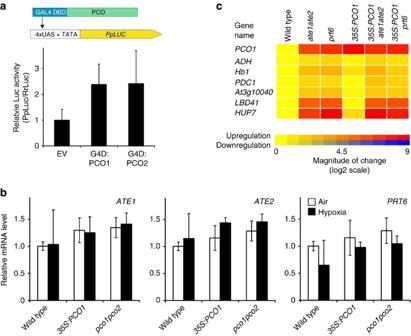Figure 4: PCOs are part of the N-end rule pathway. (a) Absence of repression of aUAS:PpLucreporter by chimeric fusions of PCO1 and PCO2 with the DNA-binding domain GAL4 (G4D) in Arabidopsis protoplasts. Data are presented as mean±s.d., one-way analysis of variance (ANOVA),n=4. (b) Overexpression ofPCO1or absence of bothPCO1andPCO2does not significantly affect the expression of genes coding for N-end rule enzymes. Expression level ofATE1,ATE2andPRT6under aerobic conditions (empty bars) and hypoxia (5% O2, 4 h) (black bars). Data, normalized to the wild type in air, are presented as mean±s.d., one-way ANOVA,n=4. (c) Differential expression of hypoxia-responsive genes inate1ate2,prt6,35S:PCO1, 35S:PCO1inate1ate2and35S:PCO1inprt6plants as compared with wild-type (reference: wild-type,n=4). Numeric expression values are shown inSupplementary Table 7. 4 ; Supplementary Table 4 ). The substantial repression of the anaerobic response by PCOs was further confirmed by a quantitative PCR (qPCR) survey on a selection of hypoxia-response genes in 35S:PCO1 and 35S:PCO2 plants ( Fig. 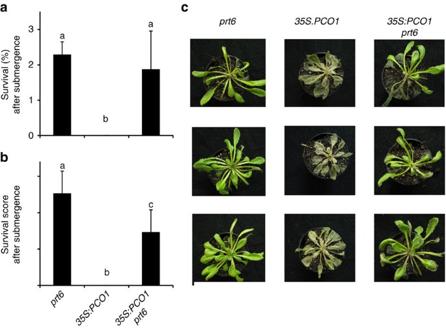Figure 5: Absence of a functional PRT6 complements the impaired flooding tolerance of 35S:PCO1. (a) Percentage ofprt6,35S:PCO1and35S:PCO1inprt6plants surviving flooding-induced hypoxia. Data are presented as mean±s.d. (n=3). Asterisks indicate statistically significant difference from the wild type (P<0.05, one-way analysis of variance (ANOVA)) (b) Tolerance score ofprt6,35S:PCO1and35S:PCO1inprt6after flooding-induced hypoxia. Data are presented as mean±s.d. (n=3). Asterisks indicate statistically significant difference from wild type (P<0.05, one-way ANOVA) (c) Phenotypes of wild type,35S:PCO1and35S:PCO1inprt6plants recovering from dark submergence (72 h). Scale bar, 2 cm. 3a ; Supplementary Table 5 ). The alteration in gene expression in PCO -overexpressing plants was accompanied by a decrease in leaf size and consequently biomass production ( Fig. 3b–d ), suggesting that an impaired ability to cope with endogenous hypoxia in certain tissues has an impact on the growth rate of the plant even when plants are growing in aerobic conditions. Figure 3: PCO1 and PCO2 redundantly repress the molecular response to hypoxia, thereby reducing tolerance to submergence. ( a ) Differential expression of hypoxia-responsive genes in PCO -overexpressing plants as compared with wild-type under aerobic, hypoxic or anoxic conditions (reference: wild-type in air, n =5). 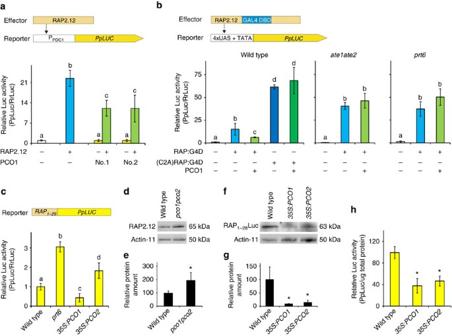Figure 6: PCO1 and PCO2 repress the activity of the hypoxic activator RAP2.12 by promoting its degradation via the N-end rule pathway. (a) Effect of PCO1 and PCO2 on RAP2.12-mediated activation of thePDC1promoter fused to aPpLucreporter in Arabidopsis protoplasts. Data are presented as mean±s.d. (n=4, the experiment was repeated three times). (b) Effect of PCO1 on RAPG4D-mediated activation of transcription in wild-type and N-end rule mutants. Data are presented as mean±s.d. (n=4, the experiment was repeated three times) (c) Effect of PCO1 on RAP2.12 stability using a fusion reporter bearing the first 28 amino acids of RAP2.12 linked to PpLuc. Data are presented as mean±s.d. (n=4, the experiment was repeated two times). Letters indicate statistically significant difference (P<0.05, one-way analysis of variance (ANOVA)). (d) Immunodetection of RAP2.12 protein in wild-type andpco1pco2plants. (e) Quantification of RAP2.12 protein via densitometry on the bands shown inSupplementary Fig. 8(means±s.d., *P<0.05,t-test,n=4). (f) Immunodetection of RAP1-18:PpLuc protein in wild-type,35S:PCO1and35S:PCO2plants. (g) Quantification of RAP1-18:PpLuc protein via densitometry on the bands shown inFig. 5d(means±s.d., *P<0.05, one-way ANOVA,n=3). (h) Quantification of Luc activity in plants expressing35S:RAP1-18:PpLucin wild type,35S:PCO1and35S:PCO2plants. Luc activity was normalized against total protein amount (means±s.d., *P<0.05, one-way ANOVA,n=4). Numeric expression values and statistical significance are shown in Supplementary Table 6 . ( b ) Phenotype of PCO1 - and PCO2 -overexpressing plants; scale bar, 2 cm. ( c ) Leaf area of wild type and 35S:PCO1 and 35S:PCO2 plants. Data are presented as mean±s.d. ( n =5). Asterisks indicate statistically significant difference from wild type ( P <0.05, one-way analysis of variance (ANOVA)). ( d ) Dry weight of wild-type and PCO -overexpressing plants. Data are presented as mean±s.d. ( n =10).Asterisks indicate statistically significant difference from wild type ( P <0.05, one-way ANOVA). ( e ) Percentage of PCO overexpressors and wild-type plants surviving flooding-induced hypoxia. Data are presented as mean±s.d. ( n =4). Asterisks indicate statistically significant difference from wild type ( P <0.05, one-way ANOVA). ( f ) Phenotypes of wild-type, 35S:PCO1 and 35S:PCO2 plants recovering from dark submergence (72 h). Scale bar, 2 cm. ( g ) Heatmap depicting the expression of hypoxia-inducible genes in pco1- , pco2- and pco1pco2 -double mutant plants as compared with the wild type under aerobic and hypoxic conditions (reference wild type in air, n =4). 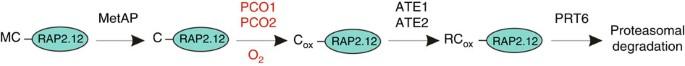Figure 7: Role of PCO1 and PCO2 in the proteasomal degradation of RAP2.12 via the N-end rule. In Arabidopsis, PCO1 and PCO2 oxidize N-terminal Cys to CSA, thereby generating an N-degron, which is recognized by arginyl transferases ATE1 and ATE2. These two enzymes add an Arg residue to the N terminus of the protein to turn it into a substrate for the E3 Ub-ligase PRT6, which covalently adds ubiquitin units. After the protein is polyubiquitinated, it is degraded by the 26S proteasome. Numeric expression values and statistical significance are shown in Supplementary Table 7 . Full size image PCO -overexpressing plants showed impaired tolerance to prolonged submergence as demonstrated by the reduced survival rate after flooding treatment ( Fig. 3e,f ). A straightforward explanation for the increased sensitivity to submergence in these plants was attributed to the inability to activate the molecular response to hypoxia as compared with the wild type, as it was actually observed when these plants were subjected to hypoxia (5% v/v O 2 ; Fig. 3a ). A similar response between wild-type and PCO -overexpressors was instead observed during anoxia (0% v/v O 2 ), indicating that molecular oxygen is required as a substrate for PCOs to counteract the induction of anaerobic genes ( Fig. 3a ). Single pco1 and pco2 knockout mutants ( Supplementary Fig. 5 ) only displayed mild alteration in the expression of typical anaerobic marker genes under normoxic conditions ( Fig. 3g ). However, when both genes were knocked out simultaneously ( pco1pco2 ), the hypoxia marker genes were significantly upregulated already under aerobic conditions ( Fig. 3g ). Moreover, on hypoxic conditions, pco1pco2 plants displayed a stronger induction of the same set of genes ( Fig. 3g , Supplementary Table 6 ). From this set of experiments, we concluded that PCOs act as oxygen-dependent repressors of the transcriptional response. PCOs function in the N-end rule pathway First, we tested whether the inhibition of the hypoxic response by PCOs could be explained by an intrinsic repression of transcription activity by these proteins. Although PCO proteins do not possess amino-acid sequences reminiscent of known repressor domains [21] , we tested their repressive activity by producing chimeric PCO1 and PCO2 fused to the DNA-binding domain of the yeast transcriptional regulator GAL4 (G4D) [22] ( Fig. 4a ). These were co-expressed in mesophyll protoplasts together with a reporter construct bearing the firefly Luciferase ( PpLuc ) gene under control of a synthetic GAL4-responsive promoter ( UAS:PpLuc) [6] . The absence of repression of PpLuc when G4D:PCO1 or G4D:PCO2 were expressed ( Fig. 4a ) confirmed that PCOs do not act as transcriptional repressors. Figure 4: PCOs are part of the N-end rule pathway. ( a ) Absence of repression of a UAS:PpLuc reporter by chimeric fusions of PCO1 and PCO2 with the DNA-binding domain GAL4 (G4D) in Arabidopsis protoplasts. Data are presented as mean±s.d., one-way analysis of variance (ANOVA), n =4. ( b ) Overexpression of PCO1 or absence of both PCO1 and PCO2 does not significantly affect the expression of genes coding for N-end rule enzymes. Expression level of ATE1 , ATE2 and PRT6 under aerobic conditions (empty bars) and hypoxia (5% O 2 , 4 h) (black bars). Data, normalized to the wild type in air, are presented as mean±s.d., one-way ANOVA, n =4. ( c ) Differential expression of hypoxia-responsive genes in ate1ate2 , prt6 , 35S:PCO1, 35S:PCO1 in ate1ate2 and 35S:PCO1 in prt6 plants as compared with wild-type (reference: wild-type, n =4). Numeric expression values are shown in Supplementary Table 7 . Full size image Albeit devoid of transcriptional activity, PCOs could still hamper the anaerobic response by indirectly enhancing the expression of N-end rule pathway key factors, such as the Arg transferases ATE1 and ATE2 or the Ub ligase PRT6 . Therefore, we conducted a real-time reverse transcriptase (RT)–qPCR analysis of the corresponding genes under aerobic or hypoxic conditions. However, no significant alteration in the messenger RNA level for each gene could be observed in plants overexpressing PCO1 or in the double-mutant pco1pco2 ( Fig. 4b ), so also this hypothesis was discarded. Alternatively, we hypothesized that PCOs may affect the activity of positive regulators of the anaerobic response by promoting their degradation via the Cys branch of the N-end rule pathway. The ERF-VII transcription factors possess a conserved Cys in the N-terminal position and have been shown to be regulated by the N-end rule pathway [6] , [11] . We first tested how PCO overexpression affects the expression of anaerobic genes that are controlled by the ERF-VII RAP2.2 or RAP2.12 in the ate1ate2 and prt6 -knockout background. Here PCO overexpression did not change the expression profile as compared with ate1ate2 and prt6 -knockout plants with normal PCO expression ( Fig. 4c , Supplementary Table 7 ). This result indicated that PCO-mediated Cys oxidation has no effect on the activity of RAP2.12 and RAP2.2 when the downstream reactions of the N-end rule pathway are not active. Consequently to the constitutive activation of the anaerobic response, the absence of a functional PRT6 increased the ability of 35S:PCO1 plants to withstand prolonged submergence in the dark ( Fig. 5 ). We therefore concluded that PCO1 and PCO2 act upstream of the N-end rule enzymes ATE and PRT. Figure 5: Absence of a functional PRT6 complements the impaired flooding tolerance of 35S:PCO1. ( a ) Percentage of prt6 , 35S:PCO1 and 35S:PCO1 in prt6 plants surviving flooding-induced hypoxia. Data are presented as mean±s.d. ( n =3). Asterisks indicate statistically significant difference from the wild type ( P <0.05, one-way analysis of variance (ANOVA)) ( b ) Tolerance score of prt6 , 35S:PCO1 and 35S:PCO1 in prt6 after flooding-induced hypoxia. Data are presented as mean±s.d. ( n =3). Asterisks indicate statistically significant difference from wild type ( P <0.05, one-way ANOVA) ( c ) Phenotypes of wild type, 35S:PCO1 and 35S:PCO1 in prt6 plants recovering from dark submergence (72 h). Scale bar, 2 cm. Full size image PCO1 and PCO2 initiate RAP2.12 proteolysis To demonstrate that PCOs are involved in controlling the activity of ERF-VII transcription factors by promoting their degradation via the N-end rule, we made use of transient transactivation assays in protoplasts. Our reporter construct consisted of the firefly Luciferase gene ( PpLuc ) under control of the Arabidopsis pyruvate decarboxylase 1 ( PDC1 ) promoter; a 35S:RAP2.12 cassette was used as activator and the effect of 35S:PCO constructs was assayed on it. Firefly luciferase activity was normalized against the one of Renilla reniformis ( RrLuc ), expressed by a 35S:RrLuc vector. Both PCOs repressed the RAP2.12-dependent activation of PpLuc ( Fig. 6a ), but did not affect the PDC1 promoter activity when RAP2.12 was not coexpressed. Similarly, PCO1 repressed the induction of gene expression mediated by RAP2.2 ( Supplementary Fig. 6 ). This effect was independent of the DNA-binding ability of RAP2.12, as demonstrated by the inhibition of the induction of the UAS:PpLuc reporter by a chimeric RAP2.12 with an additional GAL4 DNA-binding domain ( RAP:G4D ; Fig. 6b ). Figure 6: PCO1 and PCO2 repress the activity of the hypoxic activator RAP2.12 by promoting its degradation via the N-end rule pathway. ( a ) Effect of PCO1 and PCO2 on RAP2.12-mediated activation of the PDC1 promoter fused to a PpLuc reporter in Arabidopsis protoplasts. Data are presented as mean±s.d. ( n =4, the experiment was repeated three times). ( b ) Effect of PCO1 on RAPG4D-mediated activation of transcription in wild-type and N-end rule mutants. Data are presented as mean±s.d. ( n =4, the experiment was repeated three times) ( c ) Effect of PCO1 on RAP2.12 stability using a fusion reporter bearing the first 28 amino acids of RAP2.12 linked to PpLuc. Data are presented as mean±s.d. ( n =4, the experiment was repeated two times). Letters indicate statistically significant difference ( P <0.05, one-way analysis of variance (ANOVA)). ( d ) Immunodetection of RAP2.12 protein in wild-type and pco1pco2 plants. ( e ) Quantification of RAP2.12 protein via densitometry on the bands shown in Supplementary Fig. 8 (means±s.d., * P <0.05, t -test, n =4). ( f ) Immunodetection of RAP1-18:PpLuc protein in wild-type, 35S:PCO1 and 35S:PCO2 plants. ( g ) Quantification of RAP1-18:PpLuc protein via densitometry on the bands shown in Fig. 5d (means±s.d., * P <0.05, one-way ANOVA, n =3). ( h ) Quantification of Luc activity in plants expressing 35S:RAP1-18:PpLuc in wild type, 35S:PCO1 and 35S:PCO2 plants. Luc activity was normalized against total protein amount (means±s.d., * P <0.05, one-way ANOVA, n =4). Full size image The involvement of the N-end rule in the repression of RAP2.12 by PCOs was further confirmed by the observation that a substitution of the N-terminal Cys with Ala in the chimeric (C2A)RAP:G4D factor enhanced PpLuc activity, owing to (C2A)RAP:G4D protein stabilization, and prevented the repression by PCO1 ( Fig. 5b ). The same was observed after expressing the regular RAP:G4D protein in protoplasts produced from plants deficient for the N-end rule [23] , [24] (single prt6 -knockout and double ate1ate2 mutant; Fig. 6b ). Considered together, our data confirm that PCO1 and PCO2 repress the activation of transcription mediated by ERF-VII proteins via oxidation of their penultimate Cys. Further evidence that the degradation of RAP2.12 promoted by PCOs depends on its N-terminal region was obtained from transient expression of a firefly luciferase C-terminally fused to the initial 28 amino acid of RAP2.12 ( RAP 1–28 :PpLuc ; Fig. 6c ). This molecular tool allowed us to evaluate RAP protein stability, rather than measuring transcriptional activity on a promoter, as in the previous experiments. Protoplasts obtained from a prt6 mutant exhibited higher luciferase activity than wild-type cells, indicating that the RAP2.12 fragment was sufficient to confer protein instability according to the N-end rule pathway ( Fig. 6c ). In addition, overexpression of PCO1 reduced the activity of RAP 1–28 :PpLuc and absence of both PCO1 and PCO2 stabilized the reporter protein, although to a lower extent than via abolishing PRT6 functionality ( Fig. 6c ). This last observation can be attributed to a possible functional redundancy of other PCO genes in promoting the degradation of C-proteins. To obtain a biochemical evidence of the role of PCO1 and PCO2 in the degradation of RAP2.12, we compared the amount of RAP2.12 protein in wild-type and pco1pco2 seedlings via immunodetection using a RAP2.12-specific antibody. Indeed, the absence of both PCO1 and PCO2 significantly increased the amount of endogenous RAP2.12 under aerobic conditions ( Fig. 6d,e and Supplementary Fig. 7 ). To further confirm that the stability of this transcription factor relies on its N-terminal consensus, we stably introduced the 35S:RAP 1–28 :PpLuc construct into wild-type, 35S:PCO1 and 35S:PCO2 backgrounds. Western blot analyses showed that overexpression of PCOs significantly reduced the amount of reporter protein ( Fig. 6f,g and Supplementary Fig. 8 ) and could account for the reduction of PpLuc activity ( Fig. 6h ). Coherently, overexpression of RAP2.12 in a pco1pco2 background caused a very similar mutant phenotype as compared with plants overexpressing a version of this transcription factor that lacks the destabilizing Cys in its N-terminal amino-acid sequence ( Supplementary Fig. 9 ) [6] . In this study we report the discovery of plant-specific enzymes, named PCOs, which are required to catalyse the oxidation of N-terminal cysteine residues in proteins using molecular oxygen as co-substrate. By doing so, PCOs generate an N-degron that ultimately leads to proteasomal degradation by the activity of ATE1, ATE2 and PRT6 and the 26S proteasome ( Fig. 7 ). Figure 7: Role of PCO1 and PCO2 in the proteasomal degradation of RAP2.12 via the N-end rule. In Arabidopsis, PCO1 and PCO2 oxidize N-terminal Cys to CSA, thereby generating an N-degron, which is recognized by arginyl transferases ATE1 and ATE2. These two enzymes add an Arg residue to the N terminus of the protein to turn it into a substrate for the E3 Ub-ligase PRT6, which covalently adds ubiquitin units. After the protein is polyubiquitinated, it is degraded by the 26S proteasome. Full size image Distinctive features of the PCO enzymes are the specific affinity for Cys in N-termini over internal or C-terminal position ( Fig. 1c ), and the incorporation of two oxygen atoms into the thiol group of cysteine to form sulphinic acid. Hu et al. [10] proposed that this same reaction occurs spontaneously in animal cells in the concomitant presence of O 2 and NO, thereby assigning a role in NO signalling to the Cys branch of the N-end rule. However, the increased stabilization of RAP2.12 protein in a pco1pco2 mutant clearly indicates the requirement of enzymatic catalysis to prompt proteolysis of Cys2 proteins in plants. Although PCO proteins catalysed CSA formation without any NO donor ( Fig. 1b ), we cannot exclude the possibility that cysteine nitrosylation could contribute to this process in vivo . The specificity of PCOs for N-terminal cysteine residues de facto excludes them as regulators of the sulphinic-acid modification of internal cysteine residues such as the one observed in peroxiredoxins [25] . Instead, it is possible to extend the list of their putative substrates to the almost 200 proteins that exhibit a Cys2 in the A. thaliana proteome [6] . Moreover, additional substrates are likely to be generated via specific proteolysis that would leave cysteine residues exposed at the N terminus. As an example of their role in plant physiology, we studied the effect of an altered expression of these enzymes with respect to the best-characterized process regulated by the C branch of the N-end rule, namely, oxygen perception. We demonstrate that, by virtue of their catalytic properties, PCO1 and PCO2 prepare ERF-VII proteins for proteasomal degradation by enhancing the generation of the N-degron in an oxygen-dependent manner ( Fig. 7 ). In this perspective, PCO1 and PCO2 act in combination with the constitutively expressed ERF-VII proteins to generate a tunable oxygen-sensing mechanism. In fact, PCOs directly link the transcriptional activity of these key regulators of the hypoxic response to the actual availability of oxygen in the cell. Moreover, being direct targets of the ERF-VII transcription factors, PCOs are also able to catalyse a rapid inactivation of the anaerobic response once oxygen tension increases again. From an evolutionary point of view, the need for enzymatic catalysis might have arisen as a mechanism to modulate the intensity of the anaerobic response, especially since uncontrolled induction was shown to put survival at stake [6] . However, the presence of PCOs already under normoxic conditions ( Fig. 2a ) suggests a fundamental role of these enzymes as constitutive repressors of the anaerobic response in air. In this perspective, PCOs and ERF-VII transcription factors mirror the oxygen sensor system in animal cells, which is constituted by prolyl-hydroxylases and the transcriptional activator HIF1-α (ref. 15 ). This observation indicates a clear convergence in the evolution of animals and plants to develop a homoeostatic system dedicated to perceive oxygen availability. To conclude, the discovery of PCO proteins widens the plethora of mechanisms that regulate protein activity, highlighting the importance of identifying additional substrates of these enzymes. Indeed, the phenotypic alterations caused by PCO overexpression ( Fig. 3b ) point out additional roles of PCOs in plant growth and development: they might control the stability or activity of Cys2 proteins involved in other pathways not directly related to the response to oxygen deficiency. Plant materials A. thaliana Columbia-0 (Col-0) was used as wild-type ecotype, as described in the figure legends. Single prt6 (N684039), pco1 (N451210) and pco2 (N116554)-knockout seeds were obtained from the European Arabidopsis Stock (uNASC). ate1ate2 -knockout seeds were obtained from E. Graciet (University of Dublin, Ireland). Growth conditions and phenotypic evaluation Seeds were sown in moist soil, stratified at 4 °C in the dark for 48 h and germinated at 22 °C day/18 °C night with a photoperiod of 8 h light and 16 h darkness. Experiments in sterile conditions were carried out with 2-week-old plants grown on vertical agar plates. Plant material for western blot comparison of wild type and pco1pco2 double was obtained from etiolated seedlings grown for 4 days in liquid MS medium supplemented with 1% sucrose. For all other experiments, 5-week-old plants were used. Low-oxygen (5% (v/v) oxygen in air) treatments were performed as described previously [26] . Flooding tolerance was assayed using three independent transgenic lines. Plants were submerged with deionized water in 15-cm-high plastic boxes and kept in the dark. Leaves were at 5 cm under the water surface. After 72 h, the water was removed from the boxes and photoperiodic conditions (8 h/16 h, light/dark) were restored. Tolerance assays were repeated at least four times by using 10–20 plants per genotype each time. Cloning of the various constructs Coding sequences (CDSs) were amplified from complementary DNA templates or expression vectors using Phusion High Fidelity DNA-polymerase (New England Biolabs). Chimeric genes (integration of the Gal4 DBD inside the RAP2.12 CDS or fusion between the first 84 bp of RAP2.12 and PpLuc ) were produced by overlapping PCR [27] . All open reading frames were cloned into pENTR/D-TOPO (Life Technologies, Darmstadt, Germany). The resulting entry vectors were recombined into destination vectors using the LR reaction mix II (Life Technologies) to obtain novel expression vectors. The pGWL7 destination vector was obtained cutting an Apa I/ Spe I fragment from pBGWL7 (ref. 28 ) and ligating it into the p2GW7 (ref. 28 ) backbone. A complete list and description of the destination vectors and primers used is provided in Supplementary Tables 8 and 9 , respectively. Protein expression and purification The CDSs of PCO1 and PCO2 were cloned into pDEST17 vector (Life Technologies) to bear a construct coding for PCOs tagged by a cleavable 6-His peptide at the N terminus. The vectors were transformed into Rosetta 2 E. coli (Novagen) cells. Protein expression was induced by the addition of 0.5 μM IPTG for 18 h. Next, the cells were harvested by centrifugation at 3,500 g for 10 min, resuspended into lysis buffer (50 mM HEPES-Na + , 300 mM NaCl, 5 mM MgCl 2 , pH 7.5) supplemented with 1 mM phenylmethylsulphonyl fluoride and lysed using an EmulsiFlex-C3 high pressure homogenizer (Avestin Inc., Ottawa, Canada). The cell lysate was then centrifuged at 20,000 g and the supernatant used was loaded onto a C 10/10 chromatography column (GE Healthcare) containing 2 ml of Talon Co 2+ resin (Clontech Laboratories Inc., Mountain View, CA, USA) equilibrated with four volumes of lysis buffer. The column was subsequently washed with 20 ml lysis buffer followed by 20 ml wash buffer (50 mM HEPES-Na + , 300 mM NaCl, 5 mM MgCl 2 , pH 7.0). Proteins were eluted with elution buffer (50 mM HEPES, 300 mM NaCl, 150 mM imidazole, 5 mM MgCl 2 , pH 7.0), quantified by BCA assay (Pierce BCA assay kit, Thermo Scientific, Rockford, USA) and the enrichment of PCO on the total protein content was verified by SDS–polyacrylamide gel electrophoresis (PAGE) Proteins were subsequently diluted in 50% glycerol and stored at −20 °C until their use in enzymatic assays [29] . CSA determination PCO activity assay was performed in 25 mM HEPES, pH 7.5 and 0.6 mM L-cysteine was used as substrate. As the importance of including and external reductant for optimal catalytic activity was shown [30] , we included 1 mM L-ascorbate in the reaction mixture. The reaction was initiated by the addition of 30 ng PCO and incubated for 10 min at 37 °C. CSA was determined by HPLC (Dionex Summit, λ ex 330 and λ em 450) after derivatization by adding 25 μl of 0.8 M borate buffer (pH 11) and 30 μl of ortho -phthalaldehyde (0.5% w/v) to 30 μl of the enzyme extract. Separation was achieved using an RP-column (Gemini 5u (C18) 110A) using an elution gradient with increasing hydrophobicity (buffer A: 0.2% (v/v) tetrahydrofuran, 20 mM sodium phosphate buffer pH 6.8; buffer B: 32.5% (v/v) methanol, 20.5% (v/v) acetonitrile, 20 mM sodium phosphate buffer pH 6.8) flow: 0.6 ml min −1 ; 0–6 min: 100% A, 20–27 min: 100% B, 27–28 min: 100% A). Oxygen consumption assay Oxygen consumption by PCO1 and PCO2 proteins was determined using an optical sensor (Presens, Germany) as a measure for enzyme activity in the same solution as used for CSA determination. Plant transformation Stable transgenic plants were obtained using the floral dip method [31] . T0 seeds were screened for kanamycin, hygromicin or phosphinotricine resistance and independent transgenic plants were identified. qRT–PCR Total RNA was isolated using a phenol-chloroform extraction protocol. Hundred milligrams FW of plant material was homogenized in 600 μl of extraction buffer (50 mM Tris–HCl pH 8.0, 300 mM NaCl, 2% SDS, 5 mM EDTA) supplemented with 10 μl of β-mercaptoethanol. KCl was added to a final concentration of 420 mM and the extract was maintained in ice for 15 min. Samples were centrifuged at 5,000 g for 5 min at 4 °C and the supernatant was collected. Four hundred and fifty microlitres of a phenol/chloroform (1:1) mixture was added. Samples were centrifuged for 5 min at 15,000 g at room temperature. The aqueous phase was recovered and an equal volume of chloroform was added and mixed. Samples were centrifuged for 5 min at 15,000 g at 4 °C and the aqueous phase was collected. Nucleic acids were precipitated with 2.5 volumes of ice-cold absolute ethanol and 1/10 volume C 2 H 3 NaO 2 3 M. After centrifugation (10 min at maximum speed, 4 °C), ethanol was removed and the dry pellet was resuspended in 50 μl of nuclease-free water. Two micrograms of total RNA was subjected to a DNase treatment (TURBO DNAse free kit; Ambion) and complementary DNA was synthetized using the SuperScript III reverse transcriptase kit (Life Technologies). Real-time PCR amplification was carried out with the ABI Prism 7900 sequence detection system (Applied Biosystems (Life Technologies), Darmstadt, Germany), using a Power SYBR-green master mix (Applied Biosystems (Life Technologies)). Ubiquitin10 ( At4G05320 ), PPR ( AT1G62930 ) and SAND family protein ( At2g28390 ) were used as housekeeping genes. Relative quantification of the expression of each individual gene was performed using the comparative threshold cycle method, as described in the ABI PRISM 7900 sequence detection system user bulletin number 2 (Applied Biosystems (Life Technologies)).Three independent transgenic lines represented by at least three plants were used and the average expression value was calculated. Microarrays Three independent PCO1 -overexpressing lines were grown in soil for 5 weeks. An identical set of plants was subsequently treated with 5% oxygen for 4 h in the dark. Total RNA from whole rosettes was extracted as described for the qRT–PCR analyses. Hybridization and scanning procedures were performed by Atlas Biolabs GmbH (Germany). Microarray analysis and data quality control were performed using RobinA [32] . Normalization of the raw data and an estimation of signal intensities were carried out using the Genechip Robust Multiarray Average methodology [33] . Microarray data related to the aerobic and hypoxic conditions were deposited in a public repository with open access (accession number GSE44342 and GSE44343, respectively). Confocal imaging For GFP imaging, leaves from independently transformed plants (2-week old) were analysed with a Leica DM6000B/SP5 confocal microscope (Leica Microsystems). Luciferase transactivation and protein stability assay Transactivation and protein stability assays were performed exploiting the Renilla reniformis and Photinus pyralis luciferase enzymes. To test the potential repression activity of PCO1 and PCO2, the respective CDSs were fused to the C terminus of the DNA-binding domain of the Saccharomyces cerevisiae GAL4 by LR recombination into the p35S-GBD-GW [33] . A four times tandem repeat UAS sequence was fused to a minimal 35S promoter and inserted into pGWL7 (ref. 28 ) to generate a reporter vector UAS:PpLuc. To evaluate the effect of PCO proteins on RAP2.12-mediated activation of the anaerobic genes, the promoter of PDC1 was cloned into pENTR-D/TOPO (Life Technologies) and recombined in pGWL7 (ref. 28 ) to generate P PDC1 :PpLuc. Similarly, effector plasmids were produced by recombining the CDS of interest from pENTR-D/TOPO into p2GW7. A RrLuc-overexpressing vector (35S:RrLuc [26] ) was used as normalization control for PpLuc reporters. Protoplasts were prepared following the protocol by Yoo et al. [34] and Ehlert et al. [35] In brief, 4-week-old wild-type or transgenic plants by incubation of 1-mm-thick leaf stripes in a solution containing 1% cellulase R-10 (Serva, Germany), 0.3% macerozyme (Serva), 0.4 M mannitol, 20 mM KCl, 20 mM MES pH 5.7, 10 mM CaCl 2 , 0.1% BSA. After 3–4 h incubation, protoplasts were filtered through a 75-μM mesh and washed twice with W5 solution (154 mM NaCl, 125 mM CaCl 2 , 5 mM KCl, 2 mM MES pH 5.7) and incubated in ice for 30 min. Protoplasts were pelletted by centrifugation (2 min at 100 g ) and resuspended in MMg solution (0.4 M mannitol, 15 mM MgCl, 4 mM MES pH 5.7). Three micrograms of each plasmid was added to 100 μl protoplast suspension (10 6 protoplasts per ml) in a 2-ml centrifuge tube. Hundred microlitres of a 40% PEG solution (0.2 M mannitol, 0.1 M CaCl 2 ) was added to each tube and the protoplast suspension was incubated 20 min at room temperature. The transformation was stopped by adding 440 μl of W5 solution. Protoplasts were pelletted by centrifugation (2 min at 100 g ), resuspended in 1 ml WI solution (0.5 M mannitol, 4 mM MES pH 5.7, 20 mM KCl, 50 mM glucose) and incubated overnight in petri plates (3 cm diameter). Later, protoplasts were pelletted by centrifugation (700 g , 2 min), flash frozen in liquid nitrogen and lysed in 100 μl 1 × passive lysis buffer (Promega). In case of stable transformants, relative luciferase activity was normalized against the total protein amount of each sample. Luciferase activities were measured using the Dual Luciferase Reporter Assay kit (Promega) with a Glomax 20/20 (Promega). SDS–PAGE and western blotting Protein samples from total tissue extracts were separated by SDS–PAGE on 10% acrylamide midigels (Bio-Rad) and then transferred onto a polyvinylidene difluoride membrane (Bio-Rad). Incubations with the antiserum and the secondary antibody conjugated to horseradish peroxidase (Agrisera) were performed following the method recommended for the ECL Plus western blotting detection system (GE Healthcare). Polyclonal anti-PpLuc (G7451 Promega) and anti-RAP2.12 (ref. 6 ) were used at 1:1,000 dilutions to detect firefly luciferase and RAP2.12, respectively. For signal normalization, a monoclonal antibody against Arabidopsis ACTIN-11 (Agrisera, AS10 702) was used at 1:3,500 dilutions. Densitometric analysis of the protein signals on the western blots was performed with the software package UVP VisionWorks LS (Ultra-Violet Products). Normalization was carried out using the ACTIN-11 signal and setting to 100 of the relative protein signal value for the wild type. Statistical analyses Significant variations between genotypes or treatments were evaluated statistically by Sigmaplot using t -test, one-way analysis of variance or two-way analysis of variance where appropriate. Mean values that were significantly different ( P <0.05) from the control or wild-type treatments are marked with an asterisk. Alternatively, mean values that are marked with a same letter do not differ. The statistical evaluation of the microarray experiments is described earlier. Accession codes: The raw data files of the microarray experiments have been deposited in the Gene Expression Omnibus database under accession codes GSE44342 and GSE44343 for aerobic and hypoxic conditions, respectively. How to cite this article: Weits, D. A. et al. Plant cysteine oxidases control the oxygen-dependent branch of the N-end-rule pathway. Nat. Commun. 5:3425 doi: 10.1038/ncomms4425 (2014).